Diminishing returns and tradeoffs constrain the laboratory optimization of an enzyme Optimization processes, such as evolution, are constrained by diminishing returns—the closer the optimum, the smaller the benefit per mutation, and by tradeoffs—improvement of one property at the cost of others. However, the magnitude and molecular basis of these parameters, and their effect on evolutionary transitions, remain unknown. Here we pursue a complete functional transition of an enzyme with a >10 9 -fold change in the enzyme’s selectivity using laboratory evolution. We observed strong diminishing returns, with the initial mutations conferring >25-fold higher improvements than later ones, and asymmetric tradeoffs whereby the gain/loss ratio of the new/old activity decreased 400-fold from the beginning of the trajectory to its end. We describe the molecular basis for these phenomena and suggest they have an important role in shaping natural proteins. These findings also suggest that the catalytic efficiency and specificity of many natural enzymes may be far from their optimum. Optimization processes, be they industrial, economical, computational or biological (evolutionary), share several common features. Graduality: each step provides an incremental improvement. Diminishing returns: the first steps yield larger improvements than the later steps [1] , [2] , meaning that the closer the process is to its optimum, the slower and less cost-effective optimization becomes. Tradeoffs: the improvement of the trait under optimization comes at the expense of other traits. These aspects of evolutionary optimization have been addressed [3] , [4] , yet our understanding of the processes that define evolutionary optimization is by no means complete. For instance, it has been shown that the first mutations have the largest impact, and diminishing returns have been observed with respect to metabolic pathways [5] , bacterial evolution [6] , population sizes [7] , mutation rates [8] and the evolution of antibiotic resistance [9] . Similarly, functional tradeoffs have been studied in the context of protein evolution [3] , [10] , [11] , [12] , yet previous works have focused on the early steps of optimization. However, exactly how diminishing returns and tradeoffs affect a complete evolutionary trajectory involving the emergence of a new catalytic activity remains unknown. Our understanding of the molecular basis for diminishing returns and tradeoffs is also limited. Finally, the potential implications of diminishing returns and tradeoffs on the existing repertoire of biomolecules, and of enzymes in particular, also remain unidentified. Overall, data and insights regarding complete functional transitions in enzymes are scarce. The starting points of natural enzymes remain mostly unknown. In addition, there is no way to reproduce the series of evolutionary intermediates that underlie the divergence of natural enzymes. Laboratory evolution (also dubbed experimental or directed evolution) can allow us to characterize every intermediate in a trajectory and thereby help us to understand the mechanisms and driving forces of evolution [13] , [14] , [15] . Such experiments have shown how new functional traits evolve, that is, by mutations increasing a latent, weak, promiscuous activity [11] , [16] , [17] , [18] , [19] . Marked switches in enzymatic functions have been achieved via laboratory evolution, whereby the catalytic efficiency of the newly evolved enzyme matched that of the starting point [20] . Although these experiments provided novel insight, they involved both random and rational (targeted) mutagenesis and/or varying substrates along the trajectory [21] . Here, we describe a complete evolutionary trajectory comprising a functional transition from a naturally occurring phosphotriesterase (PTE) from Pseudomonas diminuta that catalyses the hydrolysis of the pesticide paraoxon with high efficiency ( k cat / K M =2.2 × 10 7 M −1 s −1 ) [22] , [23] , to an arylesterase that catalyses the hydrolysis of 2-naphthyl hexanoate (2NH; Fig. 1 ). Although the original (PTE) and new (arylesterase) enzymes catalyse hydrolysis, the reactions differ in the bond that is hydrolysed (P–O versus C–O), the shape and binding orientation of the substrates, and the geometry of the substrates (tetrahedral versus planar) and transition states (TSs) (pentavalent versus tetrahedral; Fig. 1 ). The laboratory evolution began from the weak, promiscuous, arylesterase activity of wild-type PTE ( k cat / K M with 2NH=4.2 × 10 2 M −1 s −1 ). Iterations of random mutagenesis and selection for variants exhibiting higher arylesterase rates led to the gradual fixation of 18 substitutions, and a highly efficient arylesterase ( k cat / K M =1.7 × 10 7 M −1 s −1 ). We isolated and characterized the intermediates of this process, and could thus describe the entire trajectory. By producing and characterizing this evolutionary trajectory, we provide a quantitative description of the magnitude of diminishing returns and tradeoffs throughout this trajectory, and also describe the molecular basis of diminishing returns and tradeoffs. 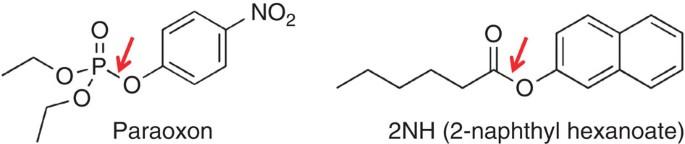Figure 1: Structures of substrates. PTE’s native substrate, paraoxon (a phosphotriester pesticide), and the promiscuous arylester 2NH that comprised the evolutionary target. Figure 1: Structures of substrates. PTE’s native substrate, paraoxon (a phosphotriester pesticide), and the promiscuous arylester 2NH that comprised the evolutionary target. Full size image Directed evolution of an arylesterase The early steps of PTE’s evolution into an arylesterase have been described previously [24] , [25] , [26] . A PTE variant with higher expression in Escherichia coli , dubbed PTE-S5, was previously evolved via random mutagenesis and screening with 2-naphthyl acetate [24] . PTE-S5 carried three mutations (Lys185Arg, Asp208Gly and Arg319Ser) compared with the wild-type PTE. These mutations improved the levels of soluble and functional enzyme in E. coli but did not modify PTE’s enzymatic activities [24] . The variant that served as our starting point for this trajectory (PTE-R0) possessed four additional substitutions compared with PTE-S5 (including two substitutions in the active site: Ile106Leu and Phe132Leu). PTE-R0 exhibited 1.7-fold higher arylesterase activity than wild-type PTE and PTE-S5, and 1.6-fold lower paraoxonase activity ( Supplementary Table S1 ). By virtue of its much higher expression levels and of its slightly higher arylesterase activity, PTE-R0 could serve as a starting point for our trajectory, because in contrast to wild-type PTE, it showed a detectable level of 2NH activity in the cell lysates. PTE-R0 was subjected to random mutagenesis and screening with 2NH to identify variants with enhanced arylesterase activity. Mutagenesis was performed in vitro by error-prone PCR. The resulting library (~10 4 transformants) was plated on agar and screened for 2NH hydrolysis using the FAST Red indicator that reacts with the released 2-naphthol product. Active colonies were subsequently grown, lysed and tested for enzymatic activity in 96-well plates. Variants that showed detectable improvements relative to the best variant from the previous round (≥1.3-fold) were isolated and used as the template for the next round of mutagenesis and screening. In rounds where multiple variants were isolated, DNA shuffling was performed to recombine beneficial mutations ( Table 1 ). The acquisition of the arylesterase activity was facilitated by chaperonin overexpression, as described previously [26] . At later stages, chaperonin coexpression was suppressed and growth temperature restored to 37 °C to promote the accumulation of compensatory, stabilizing mutations (rounds 3 and 10–12; Table 1 ). Table 1 Summary of experimental conditions in each round of the evolution Full size table The first 14 rounds of mutagenesis and screening showed detectable and reproducible improvements in the rate of 2NH hydrolysis, as measured in crude cell lysates ( Fig. 2a ). By the fifteenth round, however, the improvement plateaued. At this stage, a high fraction of the library variants exhibited high activity, but none appeared better than the starting point (>1.3-fold 2NH activity compared with R14). We therefore relaxed the selection pressure, and during the fifteenth round, 190 of the screened variants that showed ≥30% activity of the starting point (the best R14 variant) were subjected to gene shuffling ( Table 1 ). However, no improved variants were found in this library. The sixteenth and seventeenth rounds behaved similarly. 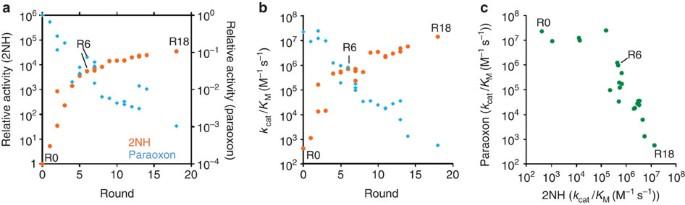Figure 2: The divergence of an arylesterase from an existing phosphotriesterase. (a) The observed gain in the evolved arylesterase activity with 2NH and the loss of the original PTE activity. The enzymatic activity in crude cell lysates is plotted. (b)kcat/KMvalues measured with purified enzyme variants (sequences and kinetic parameters are provided inTables 2,3). (c)A tradeoff plot of the arylesterase (2NH) versus the original, paraoxonase activity. By the eighteenth round, the best variants showed only twofold higher 2NH hydrolysis rates than the best R14 variant, although they carried four additional mutations ( Table 2 and Fig. 2a ). Thus, the weaker selection pressure (taking variants with lower activity than the starting point) enabled us to accumulate neutral and slightly advantageous mutations that ultimately led to detectable, albeit small improvements. Figure 2: The divergence of an arylesterase from an existing phosphotriesterase. ( a ) The observed gain in the evolved arylesterase activity with 2NH and the loss of the original PTE activity. The enzymatic activity in crude cell lysates is plotted. ( b ) k cat / K M values measured with purified enzyme variants (sequences and kinetic parameters are provided in Tables 2 , 3). ( c ) A tradeoff plot of the arylesterase (2NH) versus the original, paraoxonase activity. Full size image Table 2 The mutations of variants. Full size table A gradual functional transition with strong diminishing returns Over 18 rounds, the evolving arylesterase activity increased gradually and smoothly, as indicated by the activity in crude cell lysates ( Fig. 2a ). This was also our screening parameter, reflecting both the specific activity (activity per enzyme molecule) and amount of folded, active enzyme. 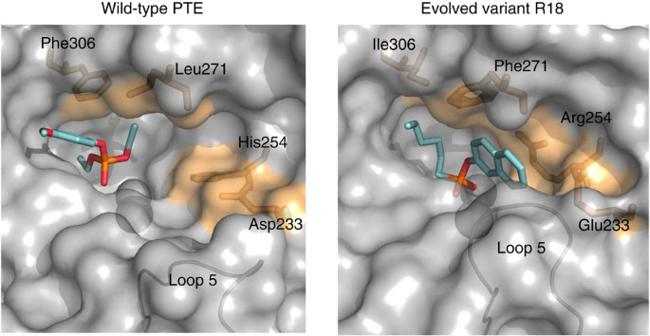Figure 3: The reshaping of the active-site cavity. Surface views of wild-type PTE’s active site with the paraoxon analogue, diethyl 4-methoxyphenyl phosphate, and that of the evolved arylesterase R18 in complex with the phosphonate analogue of 2NH’s TS (Protein Data Bank accession code:4E3T). The wild-type complex was modelled by superimposing the >90% identical structure of the PTE fromAgrobacterium radiobactercomplexed with diethyl 4-methoxyphenyl phosphate (Protein Data Bank accession code:2R1N)23,27with the structure of PTE (Protein Data Bank accession code:1DPM). The four first-shell mutations are depicted as sticks. The position of the C-main chain of loop 5 is shown, and the active-site metals are illustrated as spheres. The kinetic parameters measured with purified variants indicated a parallel increase in the arylesterase activity ( k cat / K M increase of 3.3 × 10 4 -fold; Table 3 and Fig. 2b ). The improvement in the arylesterase activity occurred gradually, and was characterized by strong diminishing returns. The early steps involved marked improvements: ~1,100-fold in the first four rounds, via four substitutions. Over the subsequent five rounds (until R9), the activity increased by another sevenfold via five substitutions. In the last rounds (R10–R18), nine more substitutions only gave a 4.4-fold higher rate. Over the entire trajectory, we observed a >25-fold decline in the return per mutation: from an increase by ~4.8-fold per substitution in the first four rounds, down to ~0.18-fold in the last eight rounds. Table 3 The kinetic parameters of variants. Full size table Asymmetric tradeoffs between the original and new activity The PTE activity was also monitored but was neither selected for nor against. Many directed evolution experiments have demonstrated that large improvements in the newly evolving function were achieved with much smaller decreases in the original function, thus resulting in bi-functional enzymes [11] . In our evolutionary experiment, however, this trend was only apparent over the first part of the trajectory. Overall, the increase in arylesterase activity was accompanied by a 4 × 10 4 -fold decrease in the k cat / K M for paraoxon, amounting to a 10 9 -fold change between the two catalytic specificities. Unlike the smooth gain in the arylesterase activity, the loss of the PTE activity was rugged ( Table 3 and Fig. 2a ). The tradeoff between the new, evolving, arylesterase and the original PTE activities was weak at the first stages as reported previously [10] , [11] , but far stronger at the later stages. Thus, the tradeoff between the evolving esterase and the original PTE activities followed a convex pattern with R6 being the point where the rate at which the original activity was lost overtook the rate at which the new activity was gained ( Fig. 2c ). By round 6, a 1,600-fold gain in the arylesterase activity traded off with a 28-fold loss in the PTE activity (57:1 gain:loss ratio). Following round 6, this trend reversed and an overall 20-fold gain in the arylesterase activity was accompanied by a ~1,400-fold loss of PTE activity (1:7 gain:loss ratio), amounting to a 400-fold reversal in the tradeoff from the first to the second half of the trajectory. Strong diminishing returns were therefore not only seen in the improvement of the new activity, but also in the level of tradeoff with the original activity. These results indicate that the specialization of enzyme function can be shaped under selection for one catalytic activity, and without negative selection against the original [20] . Specialization, however, only occurred during the later rounds, was accompanied by relatively small improvements in the newly evolved function, and was incomplete (R18 exhibited a clear vestige of the original paraoxonase activity; k cat / K M =560 M −1 s −1 ). The molecular basis of diminishing returns and asymmetric tradeoffs To investigate the molecular basis of the strong diminishing returns and asymmetric tradeoffs, a structure of R18 with a bound phosphonate TS analogue of 2NH was solved (1.65 Å resolution; Supplementary Fig. S1 , Supplementary Table S2 and Supplementary Methods ). Although as expected, the overall architecture of wild-type PTE was retained (RMSD (root-mean-square deviation)) for R18’s C-α atoms is 0.6 Å), the substrate-binding cavity of R18 was completely reshaped ( Fig. 3 ). Surprisingly, given the substantial change in this cavity, only 4 of 18 mutations are located within the enzyme’s active site (first shell), with a further 8 mutations in the active-site periphery (second shell) and the remaining 6 mutations on the enzyme’s surface (third shell). Notably, the inner-shell mutations were accumulated in the first rounds and outer-shell mutations in the later rounds ( Table 2 and Fig. 4a ). The chronological order of accumulation of the mutations from the first to outer shells relates to the strong diminishing returns of the arylesterase activity. The effects of the mutations could be classified as follows: Figure 3: The reshaping of the active-site cavity. Surface views of wild-type PTE’s active site with the paraoxon analogue, diethyl 4-methoxyphenyl phosphate, and that of the evolved arylesterase R18 in complex with the phosphonate analogue of 2NH’s TS (Protein Data Bank accession code: 4E3T ). The wild-type complex was modelled by superimposing the >90% identical structure of the PTE from Agrobacterium radiobacter complexed with diethyl 4-methoxyphenyl phosphate (Protein Data Bank accession code: 2R1N ) [23] , [27] with the structure of PTE (Protein Data Bank accession code: 1DPM ). The four first-shell mutations are depicted as sticks. The position of the C-main chain of loop 5 is shown, and the active-site metals are illustrated as spheres. 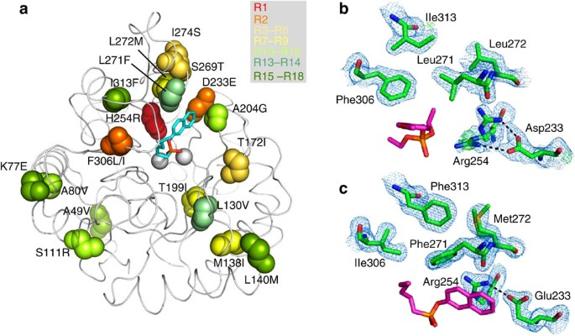Figure 4: The molecular basis of diminishing returns. (a) Backbone diagram of the evolved arylesterase (PTE-R18) with the bound 2NH TS analogue (as sticks). The substitutions underlying R18’s divergence are depicted as spheres. The colour scheme corresponding to their order of appearance is red (early), orange (intermediate) to green (late). (b) The active site of wild-type PTE-Arg254 with diethyl 4-methoxyphenyl phosphate (in magenta sticks; Protein Data Bank accession code:1QW7). Note the two rotamers of Arg25428. (c) The active site of the evolved arylesterase with the 2NH TS analogue (in magenta sticks). Arg254 adopts a single rotamer. Full size image Figure 4: The molecular basis of diminishing returns. ( a ) Backbone diagram of the evolved arylesterase (PTE-R18) with the bound 2NH TS analogue (as sticks). The substitutions underlying R18’s divergence are depicted as spheres. The colour scheme corresponding to their order of appearance is red (early), orange (intermediate) to green (late). ( b ) The active site of wild-type PTE-Arg254 with diethyl 4-methoxyphenyl phosphate (in magenta sticks; Protein Data Bank accession code: 1QW7 ). Note the two rotamers of Arg254 [28] . ( c ) The active site of the evolved arylesterase with the 2NH TS analogue (in magenta sticks). Arg254 adopts a single rotamer. Full size image (i) A key leaving group stabilizing substitution : the His254Arg mutation that was selected in R1 (2.6-fold increase in arylesterase activity) appears to be the centrepiece around which this trajectory evolved. In R18, Arg254’s side chain is positioned to stabilize the negative charge on the napthoxide leaving group by direct electrostatic interaction, and/or cation–π interactions ( Supplementary Fig. S2 ). Indeed, reversion of Arg254 to histidine in the R18 variant resulted in a >10 4 -fold reduction in the arylesterase activity, but only a fourfold reduction in the PTE activity ( Table 3 ). The Brønsted plots for both R18’s and R0’s arylesterase activity exhibit a slope of near-zero for substrates with leaving group p K a values ≥7.5, indicating that the rate-limiting step did not change throughout the trajectory ( Supplementary Fig. S3 ). In the subsequent rounds, second-shell substitutions had a role in refining the catalytic potential of Arg254 (see (iii)). (ii) Substitutions that reshaped the substrate-binding cavity : the acyl side-chain pocket of R18 was reshaped by the Phe306Leu substitution in round 2 (increasing the arylesterase activity by 12-fold) and subsequently the Leu306Ile mutation in round 7. These changes elongated the cavity. The pocket was then narrowed by the Leu271Phe mutation in round 13 ( Fig. 3 ). The reshaping of this active-site pocket is manifested in the acyl chain length preference changing from 2 to 4 in PTE-R0 to 4–6 in PTE-R18 ( Supplementary Fig. S4 ). Rearrangement of loop 5 also reshaped the active-site cleft: in R18, the tip of loop 5 is shifted 5.6 Å outwards, relative to wild-type PTE ( Fig. 3 ). It appears that a number of mutations, including Thr172Ile, Thr199Ile and Ala204Gly, have stabilized the new loop conformation. (iii) Reinforcing mutations : the molecular basis for the diminishing returns observed in this trajectory can be explained by a category of second- and third-shell substitutions that we termed reinforcing mutations. These substitutions are positioned to stabilize the geometry of the first-shell mutations, particularly Arg254. When incorporated into wild-type PTE, Arg254 adopts two rotamers, one of which sterically blocks entrance of the new substrate into the active site, whereas the other is ideally positioned to stabilize the developing negative charge on the leaving group in the TS of the reaction ( Fig. 4b ). However, only one Arg254 conformer is observed in the R18 structure, where we observe that a network of stabilizing interactions has arisen around the productive, bent, geometry ( Fig. 4c ). Asp233Glu from round 2 appears to be the primary reinforcing mutation, only forming a H-bond with Arg254 in its bent conformation. This is confirmed by the strong epistatic interaction between these mutations: the Asp233Glu mutation resulted in a 160-fold increase in arylesterase activity in the presence of Arg254 (R1), but only a 2.3-fold increase in the presence of His254 (R0; Table 3 ). After Glu233, several other mutations appear to have added robustness to this geometry, with the backbone carbonyl of Leu271Phe (round 13) also H-bonding to Arg254 in its bent form. Several second-shell mutations were located around Arg254, including Ser269Thr (round 5), Leu272Met (round 9) and Ile313Phe (round 18). Although the precise roles of these mutations remain unclear, they are likely to affect the conformation of either Arg254 and/or of Ile/Leu306 ( Fig. 4 ). Reinforcement is seen in the tolerance of R18 to the Glu233Asp reversion mutation; when reverted to Asp233 in PTE-R2, a 160-fold reduction in arylesterase activity is observed, but when the same reversion is performed in PTE-R18 the loss in arylesterase activity is only fivefold, implying that its stabilizing role has, at least partially, been reinforced by other mutations that accumulated later in the trajectory. Several other mutations accumulated around the active site, and are located on the opposite side of position 254. These include Met138Ile (round 7), Leu130Val (round 13) and Leu140Met (round 18). Currently, their roles in switching PTE’s catalytic activity remain unclear, but the improvements in 2NHase activity by these mutations are relatively small (<1.6-fold). (iv) Compensatory mutations : the third-shell substitutions mostly appeared during rounds of evolution in which GroEL/ES overexpression was not applied as well as the neutral drift rounds (R15–R18). They primarily comprise compensatory, global-suppressor mutations that compensate for the loss of stability associated with the first- and second-shell mutations that reshaped PTE’s active site [29] , [30] . These include Ile274Ser (round 3), Ala80Val (round 10), Ser111Arg, Ala204Gly (round 11), Ala49Val and Lys77Glu (round 18). These mutations have no effect on the catalytic specificity ( k cat / K M ). They do, however, affect the levels of soluble enzyme in the absence of GroEL/ES overexpression. For example, round 10 to round 12 were performed without GroEL overexpression ( Table 1 ). Three mutations that are distant from the active site (Ala80Val, Ser111Arg and Ala204Gly) accumulated during these rounds. The k cat / K M value of the variants carrying these mutations with 2NH remained unchanged ( Table 3 ), yet the enzymatic activity in crude cell lysates increased. The detailed characterization of these compensatory mutations will be published elsewhere. Most of these compensatory substitutions accumulated in the final rounds, thereby explaining the low return per substitution that underlined the final stages of this trajectory. The convex tradeoff function is a result of the bi-functional nature of the evolutionary intermediates. Best represented by R6, these intermediates are efficient enzymes for both the original and the new activities ( k cat / K M of ~10 6 M −1 s −1 ). This bi-functionality may relate to the conformational plasticity of these intermediates [31] , as seen in the coexistence of the two different conformers of Arg254 described above ( Fig. 4 ). In its extended conformation, Arg254 is known to aid substrate binding during the PTE reaction [26] , but sterically prohibits the arylester entering the active site. In contrast, in its bent conformation, Arg254 provides the key electrostatic interaction in the new arylesterase catalytic mechanism ( Supplementary Fig. S5 ). Therefore, while the starting and end points of the trajectory exhibit a single active-site conformation, specialized for a single reaction, the unstabilized active sites of the intermediates are able to interconvert between two geometries. Beside the changes in the shape of active site, metal coordination changes have been observed. We also solved a structure of R18 with bound cacodylate, an analogue of the phosphodiester product of paraoxon hydrolysis, (1.50 Å resolution), and a structure of R18 in the absence of any ligand (1.85 Å). The binuclear metal ion centre of PTE at the active site (α- and β-sites) catalyses hydrolysis by stabilizing both the hydroxide nucleophile and the developing negative charge on the TS [23] , [28] , [32] , [33] . The metal ion centre also involves the carboxylation of a lysine residue [34] . Both metal ions are seen in the available PTE structures, including engineered mutants [35] , [36] . However, the ligand-free structure of R18 was found to have a barely occupied β-site, a partially filled α-site and a previously unseen observed γ-site ( Supplementary Fig. S6 and Supplementary Fig. S7 ). Metal-ion reconstitution experiments indicated that complete reactivation of apo-R18 is achieved at 2:1 Zn 2+ :enzyme stoichiometry ( Supplementary Fig. S8 ). This suggests that the original binuclear state remains the catalytically relevant form. Indeed, the binuclear centre is seen in the structures of R18 with bound TS analogue and cacodylate: the occupancy of Zn 2+ at the β-site is significantly higher in these structures, and at a comparable level to the occupancy of the ligand. In other words, the same binuclear active-site functions in R18 as in PTE, but in R18 it seems to be dependent on substrate binding ( Supplementary Fig. S7 ). Indeed, R18 loses activity much more rapidly than R0 in metal-ion-free buffer ( Supplementary Fig. S9 ). The evolution of PTE into R18 has therefore resulted in the metal-ion-binding affinity being significantly weakened, and in the emergence of the γ-site, the role of which in the arylesterase activity remains to be understood. The complete transition in enzyme activity, a 10 9 -fold shift in the PTE/arylesterase catalytic specificities, sheds light on the molecular basis of the diminishing returns and asymmetric tradeoffs that underlined this functional switch. Although we do not exclude the possibility of alternative trajectories that lead to the same outcome (arylesterase), which may exhibit different dynamics, we surmise that these features are general. As diminishing returns are observed in various biological systems [5] , [6] , [7] , [8] , [9] , this phenomenon would be an inherent property of all optimization/evolutionary processes. Either in nature or in the laboratory, evolution selects variants from the population that best meet the selection criteria. Naturally, few mutational solutions are available that give large improvements, and these seem to be exhausted within the first few generations. The diminishing returns seem to relate to the fact that over the 18 rounds, the mutations appear to radiate outwards from the first mutations within the active site, to the later mutations stabilizing the enzyme or reinforcing the effects of the early ones. Only 4 out of 18 mutations were located in the first shell of the active site and directly contact the substrates, and 3 out of these 4 mutations appeared in the first two rounds of evolution. The structural analysis indicates the later mutations reinforce the effects of the early ones. The proposed reinforcement model explains the frequent observation from directed evolution experiments that second- and third-shell mutations improve enzyme and protein functions [10] , [21] , [37] , [38] , [39] . Compensatory mutations that alleviate the stability losses imposed by the active-site mutations also belong to this category [29] , [30] , [40] , [41] . They appeared at positions distant from the active site (third shell, primarily) and provide further support for the role of distant mutations in the evolution of new protein functions. The strong diminishing returns and asymmetric tradeoff observed in the evolutionary optimization of our laboratory-evolved arylesterase illustrate how difficult it is to achieve full optimization of a trait such as catalytic specificity and provide a molecular explanation for the sub-optimal kinetic parameters and broad specificity observed in many naturally evolved enzymes. Our in vitro evolution protocol yielded one mutation per gene per generation, and the most active variant from every round was selected. It thereby resulted in the complete fixation of mutations in the selected variants, regardless of the level of improvement these mutations provided. In other words, mutations were fixed at a constant pace of one per generation (round), so long as they provided a selective advantage, but irrespective of their fitness gain (selection coefficient) and population size. In nature, the selection pressures acting to refine enzyme activity are far more complex. Foremost, the likelihood of fixation of a mutation is proportional to its fitness gain and also depends on population size. Mutations that provide relatively small gains, as observed here from round 5 thereafter, may require many generations to fixate, or may never fixate, particularly within small populations [42] , [43] . Thus, the final refinement stages of enzymes whose contribution to overall organismal fitness is small and/or transitory can be extremely slow, or may never occur. Indeed, a recent bioinformatics study showed the average k cat / K M value of enzymes in secondary metabolism (7 × 10 4 M −1 s −1 ) is ca. an order of magnitude lower than enzymes in primary metabolism, and the average k cat value is >30-fold lower [44] . Overall, enzymes in secondary and specialized metabolism seem multifunctional and poorly specialized, in accordance with their weak and transient contribution to survival and growth rates [45] . Similarly, the asymmetric tradeoff that results in high-catalytic specificity for the arylesterase function only appears after round 14 (at which point the arylesterase becomes ≥1,000-fold higher than PTE activity). A growing body of evidence suggests that many enzymes exhibit broad catalytic specificity and/or promiscuity [11] , [17] , particularly enzymes in secondary metabolism [44] , [45] , [46] , [47] , [48] . Broad specificity may therefore relate to the recent divergence of secondary and specialized metabolism enzymes relative to primary metabolic enzymes, as well as the intensity of selection being weaker than it is for enzymes in primary metabolism [45] , [49] . For example, 37% of E. coli ’s enzymes catalyse more than one reaction in vivo , and they catalyse 65% of E. coli metabolic reactions [49] . The specialization appears to be related to the metabolic context—essential transformations that proceed with high flux and require more regulation [49] . It is therefore likely that many proteins, and in particular enzymes of specialized metabolic pathways, are far from their functional optimum and could be readily improved by means of laboratory evolution [50] . Materials 2NH and paraoxon were purchased from Sigma. The TS analogue of 2NH hexylphosphonate 2-naphthyl ester was synthesized based on previously published procedures [51] . Briefly, the di-2-naphthyl ester was synthesized by reacting hexylphosphonic dichloridate with 2-naphthol in dichloromethane using triethylamine as base. The reaction mixture was extracted with bicarbonate, diluted hydrochloric acid and brine. The solvent was evaporated, and the crude diester product was dissolved in acetonitrile and hydrolysed by addition of two equivalents of sodium hydroxide (2.5 h at room temperature). The solvent was evaporated, and the residual solid was dissolved in water. The released 2-naphthol was extracted into dichloromethane by mild acidification, followed by addition of 5 N HCl to extract the phosponate monoester product. The solvent was removed and the product was dissolved in water plus ammonium hydroxide. The solution was lyophilized and the resulting ammonium salt was purified by recrystallization from acetonitrile-ether-hexane. Cloning and library construction PTE genes were cloned with Nco I and Hind III sites into pET-strep [26] vector to express the strep-tag–PTE fusion protein for the evolution experiment and purification for the enzyme kinetics and stability assay. For crystallization, PTE-R18 was cloned into a modified pET32-trx vector and expressed without the tag. The modified expression vectors pET-T72, which carried two mutations in T7 promoter region (A-6T and A-16C), and pET-T74, which carried four mutations (A-6T, T-8A, A-10T and A-16C), were created by site directed mutagenesis. PTE libraries were generated by random mutagenesis with error-prone PCR using the ‘wobble’ base analogues dPTP and 8-oxo-dGTP (TriLink) and the DNA shuffling method. The first 20 PCR cycles with primers flanking the cloned genes were performed with Taq polymerase (Bioline) in 50 μl reactions using 1 ng of plasmid template, with 1 μM dPTP, 20 μM 8-oxo-dGTP and 0.25 mM of each of the four standard dNTPs. The PCR products were treated with Dpn I to digest the template plasmid, purified and then used as a template (20 ng per 50 μl reaction) for another 20 PCR cycles with nesting primers and Bio Taq polymerase (Bioline). The product of this final PCR was purified, digested with restriction enzymes Nco I and Hind III (NEB, 3 h at 37 °C) and ligated into one of the modified pET vectors as described above. This protocol created libraries carrying an average two to three nucleotide substitutions per gene with high reproducibility. Directed evolution Gene libraries were transformed into E. coli BL21 (DE3) cells carrying the pGro7 plasmids encoding the GroEL/ES chaperonin. Transformed cells were plated on LB agar plates with amp (100 μg ml −1 ampicillin), cam (34 μg ml −1 chloramphenicol) and 0.2% glucose and incubated overnight. The colonies were replicated using a velvet cloth to LB agar–amp–cam containing 100 μM ZnCl 2 , 1 mM isopropyl-β- D -thiogalactoside and 0.2% arabinose (for overexpression of GroEL/ES) or 0.2% glucose (suppression of GroEL/ES). Subsequently, top agar (0.5% agar in 100 mM Tris–HCl pH 7.5) containing 50 μM 2NH and 200 μM FAST Red (Sigma) was layered. About 3,000–5,000 colonies were screened using FAST Red in each round. Subsequently, ~540 colonies (six 96-well plates) showing the fastest development of red colour were picked from the replica plates, grown in 96-well plates and assayed for 2NH hydrolysis. Thirty variants that showed the highest 2NH hydrolase activity were picked and streaked onto LB agar–amp–cam. Three individual colonies from each variant were picked and their activities with 2NH were retested. Variants that showed ≥1.3-fold higher 2NH activity than the starting point (the best variant from the previous round) were recognized as positives. Paraoxon hydrolysis for variants was also recorded but was not taken into consideration for choosing the templates for the next round. The experimental conditions such as the mutagenesis protocol and the selection conditions (overexpression of GroEL/ES, growth temperature, promoter strength and so on) were varied in each round to maintain the screen’s dynamic range such that improved variants could be identified. When multiple variants were identified as positives, gene shuffling (homologous recombination in vitro ) was used to create the next-generation library. Enzyme purification To determine kinetic parameters, the PTE variants were purified using strep-tactin affinity columns (IBA) using the manufacturer’s protocol. The buffer of the eluted proteins was exchanged with 100 mM Tris-HCl pH 7.5, and the samples were concentrated, using Vivaspin centrifugal ultrafiltration (Satorius Stedim Biotech). For crystallization, PTE-R18 was expressed without the strep-tag, and purified by DEAE sepharose ion-exchange chromatography (GE Healthcare) followed by SP sepharose ion-exchange chromatography (GE Healthcare) and Superdex 200 size-exclusion chromatography (GE Healthcare). Enzyme kinetics Initial velocities ( v 0 ) were determined at 12 different substrate concentrations (2–2,000 μM) in 100 mM Tris-HCl pH 7.5, 100 μM ZnCl 2 and 0.02% Triton X-100. Hydrolysis rates were monitored using a microplate reader by following product formation at 500 nm for 2NH (in the presence of 2 mM FAST Red) and at 405 nm for paraoxon. K M and k cat were determined by fitting the initial rates of the Michaelis–Menten model ( v 0 = k cat [ E ] 0 [ S ] 0 /( K M +[ S ] 0 )) using KaleidaGraph (Synergy Software). The rates of enzymatic hydrolyses of the different phenol esters were determined with 4-nitrophenyl acetate (p K a of the phenol leaving group=7.14), 4-acetoxy benzaldehyde (7.66), 4-cyanophenyl acetate (7.95), 4-acetoxy acetophenone (8.05), 3-nitrophenyl acetate (8.39), 4-acetoxy methyl benzoate (8.47), 3-cyanophenyl acetate (8.61), 3-fluorophenyl acetate (9.28), phenyl acetate (10), 4-methyl phenyl acetate (10.2), 4-methoxy phenyl acetate (10.29) and 3,4 dimethyl phenyl acetate (10.34). Detailed information about these substrates and assay wavelengths is provided in Vanhooke et al. [27] Zinc ion titration PTE variants (20 μM) in 20 mM HEPES (pH 7.5) were incubated for 24 h at 4 °C in a solution with 5 mM of EDTA and 5 mM 1,10-phenanthroline. The chelators were removed by passing the mixture through an Econo-Pac 10DG gel filtration column (10 ml column volume, Bio-Rad) that was equilibrated by sequential passages of Chelex-treated 50 mM HEPES (pH 8.5). The resulting metal-free, apoenzyme (as indicated by complete loss of activity, 1 μM,) was incubated with freshly prepared solutions of ZnCl 2 at various concentrations (0.1–20 μM) in 50 mM HEPES pH 8.0 for 48 h at room temperature. The enzyme solution was diluted and the recovered catalytic activity was measured with 2NH (200 μM) and paraoxon (200 μM). Zinc ion dissociation The apoenzymes (20 μM) were reconstituted with freshly prepared 1 mM of ZnCl 2 and incubated for 48 h at 4 °C. And an excess of Zn 2+ ions was removed by passing the mixture through an Econo-Pac 10DG (Bio-Rad) gel filtration column that was equilibrated with Chelex-treated 50 mM HEPES (pH 7.5). The enzyme was diluted to 1 μM and dialysed into 50 mM HEPES, 100 mM NaCl (pH 6.5). The samples were taken from the dialysis bag, diluted, and the enzymatic activities of paraoxon and 2NH were measured every hour. Crystallization For crystallization, PTE-R18 was purified via cation exchange chromatography (Resource S column, 50 mM MES pH 6.0) and gel filtration (25 mM HEPES pH 8.0, 50 mM NaCl). Crystals were grown at pH 6.5 (50 mM MES) using 30% MPD and 2% PEG 8K as precipitants. Crystals of R18 in complex with cacodylate were grown in identical conditions, with the exception that 50 mM Na-Cacodylate was used as a buffer instead of MES. The concentration of MPD was increased to 40% for the use as a cryoprotectant during flash cooling of the crystals under a stream of nitrogen gas (100 K). For crystal soaking experiments, 10 mM hexylphosphonate 2-naphthyl ester was included in the cryobuffer and crystals were soaked for 10 min. Diffraction data were collected from beamline 14–4 at the European Synchrotron Radiation Facility at a wavelength of 0.9793 Å, or beamline 23–2 at a wavelength of 0.8726 Å. Data were integrated using the XDS package [52] and scaled using the program SCALA [53] . Data collection statistics are shown in Supplementary Table S2 . Difference Fourier maps were used to confirm the mutations identified by sequencing of R18 and the presence of the ligands, hexylphosphonate 2-naphthyl ester and cacodylate. The mutated residues and the ligand were altered accordingly in our models, and solvent and other conformational differences from the starting model were remodelled using Coot [54] . Refinement was performed with phenix.refine [55] . Five percent of the reflections were omitted from the refinement for the purpose of cross-validation. Analysis of the structure of the H254R mutant of PTE was performed using deposited structure factors and coordinates obtained from the Protein Data Bank (accession code: 1QW7 ) [56] . How to cite this article: Tokuriki, N. et al. Diminishing returns and tradeoffs constrain the laboratory optimization of an enzyme. Nat. Commun. 3:1257 doi: 10.1038/ncomms2246 (2012).